Involvement of PGC-1α in the formation and maintenance of neuronal dendritic spines The formation, maintenance and reorganization of synapses are critical for brain development and the responses of neuronal circuits to environmental challenges. Here we describe a novel role for peroxisome proliferator-activated receptor γ co-activator 1α, a master regulator of mitochondrial biogenesis, in the formation and maintenance of dendritic spines in hippocampal neurons. In cultured hippocampal neurons, proliferator-activated receptor γ co-activator 1α overexpression increases dendritic spines and enhances the molecular differentiation of synapses, whereas knockdown of proliferator-activated receptor γ co-activator 1α inhibits spinogenesis and synaptogenesis. Proliferator-activated receptor γ co-activator 1α knockdown also reduces the density of dendritic spines in hippocampal dentate granule neurons in vivo. We further show that brain-derived neurotrophic factor stimulates proliferator-activated receptor γ co-activator-1α-dependent mitochondrial biogenesis by activating extracellular signal-regulated kinases and cyclic AMP response element-binding protein. Proliferator-activated receptor γ co-activator-1α knockdown inhibits brain-derived neurotrophic factor-induced dendritic spine formation without affecting expression and activation of the brain-derived neurotrophic factor receptor tyrosine receptor kinase B. Our findings suggest that proliferator-activated receptor γ co-activator-1α and mitochondrial biogenesis have important roles in the formation and maintenance of hippocampal dendritic spines and synapses. Mitochondrial biogenesis, the growth and division of pre-existing mitochondria, is a process requiring the spatiotemporally coordinated synthesis of proteins encoded by the nuclear and mitochondrial genomes [1] . Peroxisome proliferator-activated receptor γ co-activator-1α (PGC-1α) has been identified as a master regulator of mitochondrial biogenesis [2] , [3] , [4] . Transcription factors that guide PGC-1α action to specific genes include nuclear receptors and nuclear respiratory factor 1 (NRF1), which controls the expression of mitochondrial proteins including cytochrome-c (cyt-c) and mitochondrial transcription factor A (TFAM), which is critical for the initiation of mitochondrial DNA (mtDNA) transcription and replication [3] , [5] . PGC-1α is expressed at high levels in mitochondria-rich cells with high-energy demands including cardiac myocytes, skeletal muscle cells and neurons [6] . PGC-1α expression is increased in response to signals that relay metabolic needs, such as exposure to cold, fasting and physical exercise [1] , [5] , [7] . An increase of PGC-1α levels is sufficient to engage cellular pathways important for energy metabolism including mitochondrial biogenesis and adaptive thermogenesis [2] , [5] , [7] . During central nervous system development, neurons are generated from proliferative neural stem cells in the process of neurogenesis. The newly generated neurons then grow axons and dendrites and form synapses to establish functional neuronal circuits. Beyond providing ATP, the evidence that mitochondria have regulatory roles in sculpting cytoarchitecture during development of nervous systems is based largely on correlational data such as changes in the location or properties of mitochondria during developmental processes [8] . A previous study suggested a role for mitochondrial dynamics in dendritic spine plasticity [9] . However, whether mitochondrial biogenesis has roles in the formation and plasticity of synapses in the developing and/or adult brain is unknown. During neuronal differentiation and maturation the number of mitochondria per cell increases, and treatment with chloramphenicol (an inhibitor of mitochondrial protein synthesis) prevents differentiation of the cells whereas oligomycin (an inhibitor of the mitochondrial ATP production) does not, suggesting that increased mitochondrial mass is required for neuronal differentiation [10] . As the energy demand of neurons increases as they become excitable and form synapses, we designed experiments to determine whether PGC-1α and mitochondrial biogenesis regulate the formation and plasticity of neural circuits. Brain-derived neurotrophic factor (BDNF) has key roles in the development, maintenance and repair of the nervous system [11] , and has emerged as an important regulator of synaptic plasticity and learning and memory [12] , [13] . BDNF has rapid effects on synaptic transmission and membrane excitability by increasing the number of docked vesicles at the active zones of synapses [14] and/or altering the activation kinetics of N -methyl- D -aspartate receptors [15] . BDNF also regulates slower cellular events involved in the formation and adaptive modification of neuronal circuits. For example, BDNF increases dendritic complexity in hippocampal dentate granule neurons [16] and increases the number of dendritic spines in CA1 pyramidal neurons [14] , [17] . BDNF and its high-affinity receptor tyrosine receptor kinase B (TrkB) are widely expressed in the developing and adult mammalian brain [18] . It was previously reported that BDNF can influence cellular energy metabolism in embryonic central nervous system neurons [19] , but it is not known if BDNF signaling affects PGC-1α and mitochondrial biogenesis, nor whether such actions of BDNF are critical for the formation and plasticity of synapses in the developing and adult brain. Here, we used molecular manipulations of PGC-1α levels to establish requirements for PGC-1α in the regulation of dendrite outgrowth and dendritic spine formation in embryonic hippocampal neurons, and in the maintenance of hippocampal dendritic spines in the adult brain. Moreover, we show that BDNF enhances dendritic spine formation, in part, by a mechanism involving upregulation of PGC-1α by the transcription factor cyclic AMP response element-binding protein (CREB). Mitochondrial biogenesis is associated with neural development When dissociated cells from E17 rat hippocampus are cultured in neuronal differentiation medium, they differentiate into neurons; subsequently, the newborn neurons grow an axon and dendrites and eventually form synapses [20] . Mitochondria in individual neurons were visualized by loading them with Mitotracker Green (mt-green) at 1 day in culture or by transfecting them with a mt-DsRed construct [21] (DsRed fused to the mitochondrial targeting sequence of cyt-c oxidase). Owing to low-transfection efficiency (~5%), the mitochondria in the neurites of individual transfected neurons are clearly visualized ( Fig. 1a ). The mitochondrial number in the neurons progressively increased as axons and dendrites grew and synapses formed ( Fig. 1a ). We also analysed the total mitochondrial mass of the neurons using mt-green (MTG) fluorescence intensity in living neurons. MTG fluorescence intensity increased by approximately eightfold between culture days 1 and 12 ( Fig. 1c ). Furthermore, cellular ATP levels (normalized to cellular protein level) increased progressively during the 12-day period in culture ( Fig. 1d ). The fold increase in mitochondrial mass was greater than the fold increase in ATP levels, which is likely due to the increased ATP utilization that occurs in neurons as they become electrically excitable and spontaneous synaptic activity occurs. The mitochondrial length frequency distribution did not change significantly, with an average mitochondrial length of ~2 μm being maintained through culture day 10 ( Fig. 1e ). Therefore, the increased mitochondrial mass as neurons grow results primarily from increased biogenesis of mitochondria, which are distributed throughout the neurites. These findings reveal an association between mitochondrial biogenesis and the active period of neurite outgrowth and synaptogenesis, suggesting a potential role for mitochondria in these developmental processes. 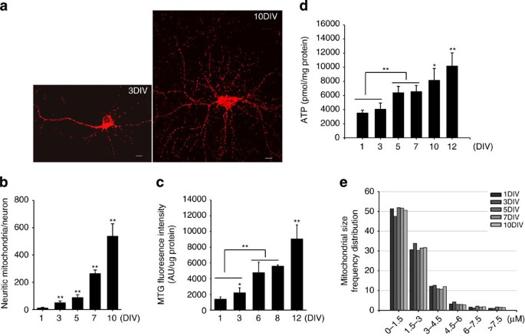Figure 1: Numbers of mitochondria increases during the differentiation and maturation of hippocampal neurons. (a) Confocal images of primary cultured hippocampal neurons at 3 and 10 days (3 DIV and 10D IV) in culture showing mt-Dsred fluorescence in individual neurons. Scale bar, 10 μm. (b) Results of counts of mitochondrial number in individual neurons at different culture days, as indicated. (c) Results of measurements of mitochondrial mass determined by mt-green fluorescence (MTG) intensity normalized to cellular protein concentration (see Methods). (d) Results of measurements of ATP concentration (normalized to cellular protein levels) at different culture days as indicated. Values are mean±s.d. (n=4–5 separate cultures). *P<0.05 and **P<0.01 (analysis of variance with Student Newman–Keulspost-hoctests). (e) The length of mitochondria in neurites was measured and the frequencies of the mitochondrial size were plotted (10–20 neurons were analysed for each condition). Figure 1: Numbers of mitochondria increases during the differentiation and maturation of hippocampal neurons. ( a ) Confocal images of primary cultured hippocampal neurons at 3 and 10 days (3 DIV and 10D IV) in culture showing mt-Dsred fluorescence in individual neurons. Scale bar, 10 μm. ( b ) Results of counts of mitochondrial number in individual neurons at different culture days, as indicated. ( c ) Results of measurements of mitochondrial mass determined by mt-green fluorescence (MTG) intensity normalized to cellular protein concentration (see Methods). ( d ) Results of measurements of ATP concentration (normalized to cellular protein levels) at different culture days as indicated. Values are mean±s.d. ( n =4–5 separate cultures). * P <0.05 and ** P <0.01 (analysis of variance with Student Newman–Keuls post-hoc tests). ( e ) The length of mitochondria in neurites was measured and the frequencies of the mitochondrial size were plotted (10–20 neurons were analysed for each condition). Full size image PGC-1α enhances dendritic spine formation and maintenance To investigate whether mitochondria are involved in regulating neural plasticity during neuronal maturation, we used molecular genetic methods to target PGC-1α, a key regulator of genes that control mitochondria biogenesis [1] , [2] , [3] , [4] , [5] . We used RNA interference (RNAi) technology to reduce PGC-1α levels in cultured hippocampal neurons. The efficacy of small interfering RNA (siRNA) in reducing PGC-1α, or oφ PGC-1α overexpression, was established by analysing PGC-1α mRNA or protein levels after infecting neurons with adenoviral constructs that express green fluorescent protein (GFP) and short-hairpin RNA (shRNA) with a scrambled sequence (Ad-GFP-Si-Con), GFP and shRNA directed against the PGC-1α mRNA (Ad-GFP-Si-PGC-1α), or GFP and PGC-1α (Ad-GFP-PGC-1α) ( Fig. 2a–d ). Neurons were co-transfected with a mt-DsRed construct in combination with constructs that express GFP-Si-Con or GFP-Si-PGC-1α or GFP-PGC-1α on culture day 5, and confocal image analysis of the neurons was performed on culture day 12 to determine the effects of PGC-1α deficiency or overexpression on mitochondria and synapses. There was a marked reduction in the number and density of mitochondria in the dendrites of neurons expressing GFP-Si-PGC-1α compared with those expressing GFP-Si-Con, whereas, in contrast, neurons overexpressing PGC-1α (GFP-PGC-1α) exhibited a significant increase in mitochondrial density in dendrites compared with control neurons ( Fig. 2e ). Quantitative analysis of mitochondria number in neurites revealed a ~30% reduction in GFP-Si-PGC-1α neurons (460.6±22.9; n =15) compared with GFP-Si-Con cells (659.6±40.2; n =15; P <0.001, Student’s t -test; Fig. 2f ). As the average mitochondrial size is smaller in GFP-Si-PGC-1α neurons (1.2±0.025 μm; n =15) compared with GFP-Si-Con cells (1.92±0.037 μm; n =15), we also quantified the dendritic mitochondrial index (mitochondrial length/dendritic length), which revealed a ~40% reduction in GFP-Si-PGC-1α neurons (0.29±0.049; n =15) compared with GFP-Si-Con cells (0.49±0.057; n =15, P <0.001, Student’s t -test; Fig. 2g ). 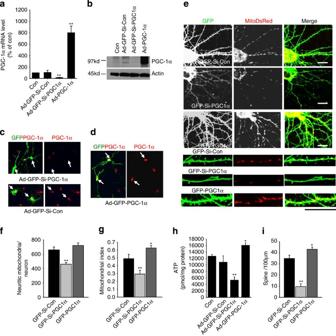Figure 2: siRNA-mediated knockdown of PGC-1α reduces mitochondrial content and dendritic spine formation in cultured hippocampal neurons. (a) Quantitative PCR using specific primers to PGC-1α demonstrates a large reduction of PGC-1α mRNA in Ad-GFP-Si-PGC-1α-infected cells and increased PGC-1α mRNA levels in Ad-GFP-PGC-1α-infected cells (48-h infection) compared with uninfected neurons and neurons expressing a scrambled shRNA (Ad-GFP-Si-Con). (b) Immunoblot analysis showing that levels of PGC-1α (~95 kd) are elevated in neurons infected with Ad-GFP-PGC-1α and are reduced in neurons infected with Ad-GFP-Si-PGC-1α compared with uninfected neurons and neurons infected with Ad-GFP-Si-Con. (c,d) Hippocampal neurons at 5 days in culture were transfected with constructs of GFP-Si- PGC-1α, GFP-Si-Con or GFP-PGC-1α, for 48 h and then fixed for immunostaining using an antibody againt PGC-1α (red). (c) GFP+cells (arrows) in GFP-Si-PGC-1α-transfected neurons exhibit little or no PGC-1α fluorescence compared with the surrounding GFP−cells or to GFP-Si-Con-transfected neurons. (d) GFP+cells (arrows) in GFP-PGC-1α-transfected neurons exhibit a stronger PGC-1α fluorescence intensity, with the PGC-1α concentrated in the nucleus, compared with surrounding GFP−cells. (e) Representative confocal images of mito-DsRed and GFP in the dendritic arbors of 12-day-old hippocampal neurons that were co-transfected with mito-DsRed and either GFP-Si-con, GFP-Si-PGC-1α or GFP-PGC-1α constructs on culture day 5. The lower panels show higher magnification of dendrites. Bars=20 μm. (f,g) Results of counts of mitochondrial numbers in the neurites of individual neurons (f) and dendritic mitochondrial density index (mitochondria/neurite length) (g) (in hippocampal neurons that were co-transfected with mito-DsRed and either GFP-Si-con or GFP-Si-PGC-1α (n=10–15 neurons analysed for each condition). Values are the mean±s.d. **P<0.01 compared with the corresponding GFP-Si-Con value (Student’st-test). (h) Results of measurements of ATP levels in 12-day-old hippocampal neurons that were infected with Ad-GFP-Si-con, Ad-GFP-Si-PGC-1α or Ad-GFP-PGC-1α on culture day 5. The results are normalized to protein concentration. Values are mean±s.d. (n=4–5 separate cultures). *P<0.05 and **P<0.01 (Student’st-test). (i) Spine density (number of spines per 100 μm) was quantified in hippocampal neurons that were transfected with either GFP-Si-con or GFP-Si-PGC-1α.n=10–15 neurons analysed for each condition. Values are the mean±s.d. **P<0.01 compared with the corresponding GFP-Si-Con value (Student’st-test). Figure 2: siRNA-mediated knockdown of PGC-1α reduces mitochondrial content and dendritic spine formation in cultured hippocampal neurons. ( a ) Quantitative PCR using specific primers to PGC-1α demonstrates a large reduction of PGC-1α mRNA in Ad-GFP-Si-PGC-1α-infected cells and increased PGC-1α mRNA levels in Ad-GFP-PGC-1α-infected cells (48-h infection) compared with uninfected neurons and neurons expressing a scrambled shRNA (Ad-GFP-Si-Con). ( b ) Immunoblot analysis showing that levels of PGC-1α (~95 kd) are elevated in neurons infected with Ad-GFP-PGC-1α and are reduced in neurons infected with Ad-GFP-Si-PGC-1α compared with uninfected neurons and neurons infected with Ad-GFP-Si-Con. ( c , d ) Hippocampal neurons at 5 days in culture were transfected with constructs of GFP-Si- PGC-1α, GFP-Si-Con or GFP-PGC-1α, for 48 h and then fixed for immunostaining using an antibody againt PGC-1α (red). ( c ) GFP + cells (arrows) in GFP-Si-PGC-1α-transfected neurons exhibit little or no PGC-1α fluorescence compared with the surrounding GFP − cells or to GFP-Si-Con-transfected neurons. ( d ) GFP + cells (arrows) in GFP-PGC-1α-transfected neurons exhibit a stronger PGC-1α fluorescence intensity, with the PGC-1α concentrated in the nucleus, compared with surrounding GFP − cells. ( e ) Representative confocal images of mito-DsRed and GFP in the dendritic arbors of 12-day-old hippocampal neurons that were co-transfected with mito-DsRed and either GFP-Si-con, GFP-Si-PGC-1α or GFP-PGC-1α constructs on culture day 5. The lower panels show higher magnification of dendrites. Bars=20 μm. ( f , g ) Results of counts of mitochondrial numbers in the neurites of individual neurons ( f ) and dendritic mitochondrial density index (mitochondria/neurite length) ( g ) (in hippocampal neurons that were co-transfected with mito-DsRed and either GFP-Si-con or GFP-Si-PGC-1α ( n =10–15 neurons analysed for each condition). Values are the mean±s.d. ** P <0.01 compared with the corresponding GFP-Si-Con value (Student’s t -test). ( h ) Results of measurements of ATP levels in 12-day-old hippocampal neurons that were infected with Ad-GFP-Si-con, Ad-GFP-Si-PGC-1α or Ad-GFP-PGC-1α on culture day 5. The results are normalized to protein concentration. Values are mean±s.d. ( n =4–5 separate cultures). * P <0.05 and ** P <0.01 (Student’s t -test). ( i ) Spine density (number of spines per 100 μm) was quantified in hippocampal neurons that were transfected with either GFP-Si-con or GFP-Si-PGC-1α. n =10–15 neurons analysed for each condition. Values are the mean±s.d. ** P <0.01 compared with the corresponding GFP-Si-Con value (Student’s t -test). Full size image As importation of mt-Dsred [21] into mitochondria is a membrane potential-dependent process, we immunostained the neurons expressing mt-Dsred with an antibody against porin (a protein located in the outer membrane of all mitochondria). The results show that all porin-immunoreactive mitochondria are also mt-Dsred positive regardless of whether PCC-1α levels are knocked down ( Supplementary Fig. S1a,b ). In addition, immunoblot analysis of porin demonstrated a significant (~40%) reduction of porin levels in neurons in which PGC-1α was knocked down compared with neurons expressing a scrambled control shRNA ( Supplementary Fig. S1c,d ). These data collectively confirm a mitochondrial mass reduction in neurons in response to PGC-1α knockdown. There was no apparent increase of mitochondrial number in neurons overexpressing PGC-1α; however, the average mitochondrial length was increased significantly in GFP-PGC-1α neurons (2.63±0.041 μm; n =15) compared with GFP-Si-Con cells (1.92±0.037 μm; n =15; P <0.01, Student’s t -test), and the dendritic mitochondrial index was ~28% greater in GFP-PGC-1α neurons (0.62±0.036; n =15) compared with GFP-Si-Con cells (0.49±0.057; n =15; P <0.001, Student’s t -test; Fig. 2f ), indicating an increase in mitochondrial mass. Next, we found that neurons in which PGC-1α was knocked down had significantly reduced ATP levels, whereas neurons overexpressing PGC-1α had elevated ATP levels, compared with control neurons ( Fig. 2h ). There was a ~55% reduction of ATP levels in Ad-GFP-Si-PGC-1α-infected neurons (5,328.1±998.4 pmol per mg protein) and a ~20% increase of ATP levels in PGC-1α-overexpressing neurons (16,088.3±783.0 pmol per mg protein) compared with uninfected neurons (12,711.8±532.4 pmol per mg protein) and neurons infected with Ad-GFP-Si-Con (10,868.9±1,952.3 pmol per mg protein). Collectively, these data indicate that mitochondrial mass and ATP levels in hippocampal neurons are dependent on PGC-1α. Examination of GFP fluorescence in dendrites revealed a marked reduction by ~75% in the density of dendritic spines in neurons expressing GFP-Si-PGC-1α (9.6±2.6 spines per 100 μm) and a significant increase by ~20% in neurons expressing GFP-PGC-1α (43.1±1.9) compared with neurons expressing GFP-Si-Con (34.9±3.0 spines per 100 μm; n =12; Fig. 2e ). Immunostaining demonstrated that immunoreactive puncta for Synapsin, a protein associated with small synaptic vesicles in presynaptic terminals [22] and PSD95, a prominent postsynaptic density scaffold protein [23] , were also markedly reduced by 67% and 71%, respectively, in neurons expressing GFP-Si-PGC-1α compared with those expressing GFP-Si-Con (PSD95, 16.5±4.3 versus 49.4±3.4 puncta per 100 μm; Synapsin I, 12.6±2.7 versus 42.9±3.0 puncta per 100 μm; n =10; Fig. 3a–c ). 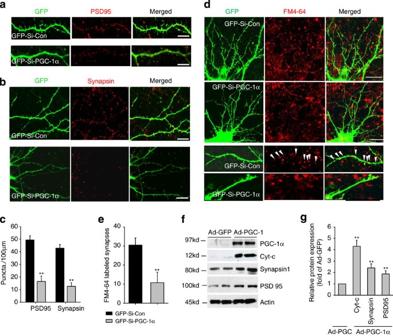Figure 3: Evidence that PGC-1α has a pivotal role in the molecular differentiation of synapses in developing hippocampal neurons. (a,b) Representative confocal images of dendritic segments at high magnification in 12-day-old neurons fixed and immunostained with PSD95 (a) or synapsin I (b) antibodies after transfecting GFP-Si-con or GFP-Si-PGC-1α constructs on culture day 5. Scale bar, 20 μm. (c) Numbers of PSD95 and Synapsin I-immunoreactive puncta (number of puncta per 100 μm;n=10–15 neurons analysed for each condition). Values are the mean±s.d. **P<0.001 compared with the corresponding GFP-Si-Con value(Student’st-test). (d) Images of hippocampal neurons at 12 days in culture that had been transfected withGFP-Si-con or GFP-Si-PGC-1α on culture day 5. Neurons were then processed for evaluation of activity-dependent uptake of the fluorescent probe FM4-64 into presynaptic terminals (see Methods). (e) FM4-64-labeled puncta (red) were quantified (number of FM4-64 puncta per 100 μm) in 10–15 neurons/culture/condition. Values are mean±s.d. (n=4–5 separate cultures). **P<0.01 (Student’st-test). (f) A representative immunoblot of PGC-1α, cyt-c, Synapsin 1, PSD95 and actin in 12-day-old hippocampal neurons that were infected with Ad-GFP or Ad-GFP-PGC-1α on culture day 5. (g) Results of densitometric analysis of blots showing cyt-c, Synapsin 1 and PSD95 protein levels (fold change compared with the value for neurons infected with Ad-GFP-Con) as in (f). Values are mean±s.d. (n=4–5 separate cultures). **P<0.01 (Student’st-test). Figure 3: Evidence that PGC-1α has a pivotal role in the molecular differentiation of synapses in developing hippocampal neurons. ( a , b ) Representative confocal images of dendritic segments at high magnification in 12-day-old neurons fixed and immunostained with PSD95 ( a ) or synapsin I ( b ) antibodies after transfecting GFP-Si-con or GFP-Si-PGC-1α constructs on culture day 5. Scale bar, 20 μm. ( c ) Numbers of PSD95 and Synapsin I-immunoreactive puncta (number of puncta per 100 μm; n =10–15 neurons analysed for each condition). Values are the mean±s.d. ** P <0.001 compared with the corresponding GFP-Si-Con value(Student’s t -test). ( d ) Images of hippocampal neurons at 12 days in culture that had been transfected withGFP-Si-con or GFP-Si-PGC-1α on culture day 5. Neurons were then processed for evaluation of activity-dependent uptake of the fluorescent probe FM4-64 into presynaptic terminals (see Methods). ( e ) FM4-64-labeled puncta (red) were quantified (number of FM4-64 puncta per 100 μm) in 10–15 neurons/culture/condition. Values are mean±s.d. ( n =4–5 separate cultures). ** P <0.01 (Student’s t -test). ( f ) A representative immunoblot of PGC-1α, cyt-c, Synapsin 1, PSD95 and actin in 12-day-old hippocampal neurons that were infected with Ad-GFP or Ad-GFP-PGC-1α on culture day 5. ( g ) Results of densitometric analysis of blots showing cyt-c, Synapsin 1 and PSD95 protein levels (fold change compared with the value for neurons infected with Ad-GFP-Con) as in ( f ). Values are mean±s.d. ( n =4–5 separate cultures). ** P <0.01 (Student’s t -test). Full size image Double immunostaining 12 DIV hippocampal neurons using antibodies against synapsin and PSD95 revealed that ~80% puncta are immunoreactive with both antibodies, indicating that these puncta represent synapses ( Supplementary Fig. S2 ). This observation indicates that the marked suppression (~75%) of dendritic spine density in neurons in which PGC-1α is knocked down reflects a reduction in synapse formation. Indeed, a similar result was obtained when functional synapses were identified by KCl-stimulated uptake of the dye FM4-64 into presynaptic terminals [24] , [25] . Seven days after transfecting 5 DIV neurons with GFP-Si-Con or GFP-Si-PGC-1α constructs, neurons were assayed for FM4-64 uptake during a 5-min period of exposure to KCl ( Fig. 3d ). Knockdown of PGC-1α caused a significant decrease in the number of synapses labeled with FM4-64 compared with neurons expressing the scrambled control shRNA ( Fig. 3d ). There was a significant reduction of the dendritic arbor quantified by measuring the overall dendritic length (by ~20%) and the dendritic complexity quantified by counting the number of dendrite bifurcations (by~30%) in GFP-Si-PGC-1α neurons compared with GFP-Si-Con neurons ( Supplementary Fig. S3 ). We further evaluated dendritic spine density in neurons at 15 DIV after knockdown of PGC-1α at 5DIV. The control neurons exhibited an increase of dendritic spine density compared with DIV 12 neurons, whereas neurons in which PGC-1α was knocked down did not exhibit a greater spine density on DIV 15 compared with DIV 12. These results indicate that significant suppression of PGC-1α expression inhibits, but does not delay dendritic spine formation. Previous studies [26] , [27] , [28] using PGC-1α null mice have demonstrated that loss of PGC-1α leads to neurodegeneration. We evaluated cell death in neurons transfected with constructs or infected with adenovirus to express either PGC-1α shRNA or scrambled shRNA and observed neither increased bright and condensed apoptotic nuclei in cells stained with Hoechst 33342 ( Supplementary Fig. S4d ), nor increased activated caspase-3 immunofluorescence or increased cleaved form of caspase-3 by immunoblot analysis in neurons expressing PGC-1α shRNA ( Supplementary Fig. S4a–c ). Therefore, the significant suppression of dendtritic spines and functional synapses after reducing PGC-1α levels is not due to neurodegeneration. We further determined whether synaptogenesis might be augmented by increasing PGC-1α levels. Neurons were infected on culture day 5 with an adenoviral vector that expresses GFP alone (Ad-GFP) or a vector that expresses GFP plus PGC-1α (Ad-GFP-PGC-1α; the efficacy of this vector in elevating PGC-1α levels was established as shown in Fig. 2a . On culture day 12, the neurons were collected for biochemical analyses to evaluate synaptogenesis. Compared with neurons infected with Ad-GFP, those infected with Ad-PGC-1α exhibited significant increases in levels of PGC-1α and the mitochondrial protein cyt-c, as well as elevated levels of Synapsin I and PSD95 ( Fig. 3f ). Thus, elevation of PGC-1α levels is sufficient to enhance mitochondrial biogenesis and molecular differentiation of synapses in hippocampal neurons. We next asked whether PGC-1α has a role in the maintenance of synapses in the adult brain. Adenoviruses (Ad-GFP-Si-PGC-1α or Ad-GFP-Si-Con) were delivered into the hippocampal dentate gyrus of 2-month-old mice via stereotaxic microinjection. After 2 weeks, coronal brain sections were prepared and GFP fluorescence was imaged revealing GFP expression in many dentate granule neurons in which the fluorescence was distributed throughout the dendritic arbors ( Fig. 4a ). The immunostaining intensity of PGC-1α in Ad-GFP-Si- PGC-1α-infected cells was much fainter than that in Ad-GFP-Si-Con-infected cells, confirming the efficacy of PGC-1α knockdown in vivo ( Fig. 4b ). For quantitative analysis, the apical dendritic arbors and segments from secondary and tertiary dendrites ( Fig. 4c ) were imaged using X25 water or X63 oil immersion objectives on a Zeiss confocal microscope. In contrast to the effects of PGC-1α knockdown in cultured hippocampal neurons, there was no significant effect of PGC-1α depletion on total apical dendrite length or the complexity of the dendritic arbor measured by counting the number of bifurcations (Ad-GFP-Si-Con versus Ad-GFP-Si-PGC-1α; length, 802±104.3 versus 745±179 μm; bifurcations 11.2±3.4 versus 9.5±2.9; 15–20 neurons analysed; Fig. 4e ). However, the granule neurons expressing Ad-GFP-Si-PGC-1α exhibited a significant reduction in dendritic spine density of ~40% (4.3±1.1 spines per 10 μm compared with 7.4±1.5 spines per 10 μm in Ad-GFP-Si-Con neurons; 15–20 neurons analysed, P <0.001, Student’s t -test; Fig. 4g ). The results indicate that transient depletion of PGC-1α in adult mature hippocampal neurons reduces the density of dentritic spines without altering the existing dendritic morphology. PGC-1α therefore has pivotal roles in synapse maintenance in the hippocampus in vivo . 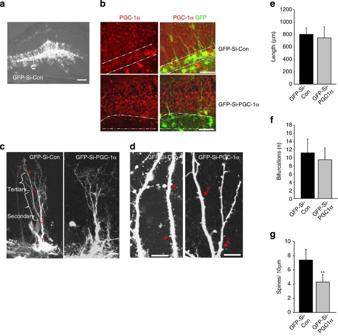Figure 4: PGC-1α is required for the maintenance of dendritic spines in adult mouse hippocampal dentate gyrus granule neurons. (a) Low-magnification images showing GFP fluorescence in neurons in the dentate gyrus. Adenoviruses that contain GFP-Si-Con or GFP-Si-PGC-1α were injected into the dentate gyrus of the hippocampus of 2-month-old male mice. Two weeks later the mice were euthanized, and brains were sectioned and confocal images of GFP fluorescence were acquired. (b) Representative confocal images showing PGC-1α immunostaining (red) and GFP (green) in the dentate gyrus of the hippocampus of mice in which granule neurons were infected with either Ad-GFP-Si-Con or Ad-GFP-Si-PGC-1α. (c,d) Representative confocal images showing dendritic trees (c) and dendritic spines (d) of neurons infected with either GFP-Si-Con or GFP-Si-PGC-1α. The dendritic spines were quantified in the secondary and tertiary segment of dendrites, which are illustrated in (b) (brackets). Scale bars in (a) 100 μm, (b) 50 μm and in (c,d) 10 μm. (e–g) Results of quantitative analysis of total dendritic length, number of bifurcations and dendritic spine density in dentate granule neurons infected with either Ad-GFP-Si-Con or Ad-GFP-Si-PGC-1α. Values are the mean±s.d. (n=5 mice; 15–20 neurons analysed per condition. **P<0.01 (Student’st-test). Figure 4: PGC-1α is required for the maintenance of dendritic spines in adult mouse hippocampal dentate gyrus granule neurons. ( a ) Low-magnification images showing GFP fluorescence in neurons in the dentate gyrus. Adenoviruses that contain GFP-Si-Con or GFP-Si-PGC-1α were injected into the dentate gyrus of the hippocampus of 2-month-old male mice. Two weeks later the mice were euthanized, and brains were sectioned and confocal images of GFP fluorescence were acquired. ( b ) Representative confocal images showing PGC-1α immunostaining (red) and GFP (green) in the dentate gyrus of the hippocampus of mice in which granule neurons were infected with either Ad-GFP-Si-Con or Ad-GFP-Si-PGC-1α. ( c , d ) Representative confocal images showing dendritic trees ( c ) and dendritic spines ( d ) of neurons infected with either GFP-Si-Con or GFP-Si-PGC-1α. The dendritic spines were quantified in the secondary and tertiary segment of dendrites, which are illustrated in ( b ) (brackets). Scale bars in ( a ) 100 μm, ( b ) 50 μm and in ( c , d ) 10 μm. ( e – g ) Results of quantitative analysis of total dendritic length, number of bifurcations and dendritic spine density in dentate granule neurons infected with either Ad-GFP-Si-Con or Ad-GFP-Si-PGC-1α. Values are the mean±s.d. ( n =5 mice; 15–20 neurons analysed per condition. ** P <0.01 (Student’s t -test). Full size image BDNF enhances PGC-1α expression and mitochondrial biogenesis It has been established that BDNF promotes neuronal differentiation and survival [11] , enhances dendrite growth, spine formation and synaptogenesis, and facilitates synaptic plasticity [16] , [17] . We next asked whether PGC-1α and mitochondrial biogenesis were involved in BDNF-induced synaptogenesis. In cultured hippocampal neurons, treatment with BDNF from culture days 5 to 12 resulted in a significant increase in the expression of PSD95 and Synapsin I in a BDNF concentration-dependent manner ( Supplementary Fig. S5 ). Strikingly, we found that the activation of the Pgc-1α promoter was increased approximately eightfold in the presence of BDNF ( Fig. 5b ) in hippocampal neurons transfected with a Pgc-1α promoter-driven luciferase reporter plasmid. In contrast, the Pgc-1α promoter with a deletion in the CRE site (CREB-binding site) exhibited reduced basal activation and was unresponsive to BDNF treatment ( Fig. 5a ). 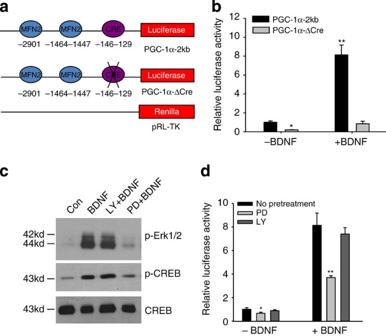Figure 5: BDNF stimulates PGC-1α promoter activity via activation of mitogen-activated protein kinases (MAPKs) and CREB. (a) Illustration of the structure of the 2-kb PGC-1α promoter linked to a firefly luciferase reporter gene harboring no mutations (PGC-1α-2 kb) or a CRE site deletion (PGC-1α-ΔCRE), and theRenillaluciferase-expressing plasmid (pRL-TK) used as an internal control. (b) Relative luciferase activity of PGC-1α-2 kb and PGC-1α-ΔCRE in neurons treated with or without BDNF for 32 h. Dual luciferase activity was measured at 48 h of transfection and the firefly luciferase activity was normalized to the level of pRL-TK Renilla luciferase activity and plotted as the fold of control (PGC-1α-2 kb, no BDNF treatment). Values are mean±s.d. *P<0.05 and **P<0.001 (n=5; analysis of variance (ANOVA) with Student Newman–Keulspost-hoctests). (c) Immunoblot analysis of phosphorylation of ERK1/2 and CREB in control and BDNF-treated neurons. Neurons were pretreated with vehicle or kinase inhibitors 30 min before exposure to BDNF (40 ng ml−1) for 30 min: MAPK inhibitor, PD980059 (PD, 20 μM); PI3K inhibitor LY 290043 (LY, 20 μM). p-ERK1/2 and p-CREB are bands in blots probed with antibodies that selectively recognize phospho-ERK1/2 and phospho-CREB; the same blots were re-probed with an antibody against total CREB (phosphorylation-independent antibody). (d) Relative luciferase activity of PGC-1α-2 kb in cells incubated under the indicated conditions. The analysis and plot are same as that described in (b). Values are mean±s.d., *P<0.05 and **P<0.001 (n=5; ANOVA with student Newman–Keulspost-hoctests). Figure 5: BDNF stimulates PGC-1α promoter activity via activation of mitogen-activated protein kinases (MAPKs) and CREB. ( a ) Illustration of the structure of the 2-kb PGC-1α promoter linked to a firefly luciferase reporter gene harboring no mutations (PGC-1α-2 kb) or a CRE site deletion (PGC-1α-ΔCRE), and the Renilla luciferase-expressing plasmid (pRL-TK) used as an internal control. ( b ) Relative luciferase activity of PGC-1α-2 kb and PGC-1α-ΔCRE in neurons treated with or without BDNF for 32 h. Dual luciferase activity was measured at 48 h of transfection and the firefly luciferase activity was normalized to the level of pRL-TK Renilla luciferase activity and plotted as the fold of control (PGC-1α-2 kb, no BDNF treatment). Values are mean±s.d. * P <0.05 and ** P <0.001 ( n =5; analysis of variance (ANOVA) with Student Newman–Keuls post-hoc tests). ( c ) Immunoblot analysis of phosphorylation of ERK1/2 and CREB in control and BDNF-treated neurons. Neurons were pretreated with vehicle or kinase inhibitors 30 min before exposure to BDNF (40 ng ml −1 ) for 30 min: MAPK inhibitor, PD980059 (PD, 20 μM); PI3K inhibitor LY 290043 (LY, 20 μM). p-ERK1/2 and p-CREB are bands in blots probed with antibodies that selectively recognize phospho-ERK1/2 and phospho-CREB; the same blots were re-probed with an antibody against total CREB (phosphorylation-independent antibody). ( d ) Relative luciferase activity of PGC-1α-2 kb in cells incubated under the indicated conditions. The analysis and plot are same as that described in ( b ). Values are mean±s.d., * P <0.05 and ** P <0.001 ( n =5; ANOVA with student Newman–Keuls post-hoc tests). Full size image Activation of the high-affinity BDNF receptor TrkB results in phosphorylation of tyrosine residues in the cytoplasmic domain of the receptor and subsequent recruitment and activation of signaling proteins that engage extracellular signal-regulated kinases (ERKs) and the phosphatidylinositol 3-kinase (PI3K)-Akt kinase pathway [29] . We found that PD98059, an inhibitor of MEK (a kinase that phosphorylates ERKs), significantly attenuated BDNF-induced Pgc-1α promoter activity, whereas the PI3K inhibitor LY98003 did not ( Fig. 5d ). Immunoblot analysis demonstrated that the phosphorylation of CREB in response to BDNF was attenuated by PD98059, but was unaffected by the PI3K inhibitors LY290043 and wortmannin ( Fig. 5c ; Supplementary Fig. S6 ). These data indicate that both ERKs and CREB mediate BDNF-induced PGC-1α promoter activity. Indeed, BDNF treatment resulted in a significant elevation of PGC-1α mRNA and protein levels within 24 h ( Fig. 6a ). Transcription factors that guide PGC-1α action to specific genes include nuclear receptors and NRF1, which controls the expression of mitochondrial proteins including cyt-c, and TFAM, which is critical for the initiation of mtDNA transcription and replication [3] , [5] . Levels of TFAM and NRF1 mRNA and protein were elevated in response to BDNF, with Nrf1 mRNA levels increasing within 4 h of stimulation with BDNF ( Fig. 6a ). 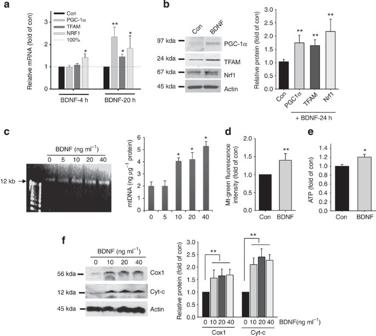Figure 6: BDNF enhances PGC-1α-mediated mitochondrial biogenesis. (a,b) Effects of BDNF on PGC-1α, NRF1 and TFAM mRNA and protein levels in cultured hippocampal neurons. Cultured hippocampal neurons (7 days in culture) were treated with 40 ng ml−1BDNF for the indicated time periods. mRNA (by quantitative PCR) and protein levels (densitometry analysis) are expressed as fold change compared with the value for vehicle-treated control neurons. Values are mean±s.d. *P<0.05, **P<0.001 (n=4; Student’st-test). (c) A representative gel showing mtDNA (left) and results of measurement of the amount of mtDNA normalized to protein concentration in cultured hippocampal neurons after treating with BDNF at indicated concentrations, or vehicle control, for 7 days (from culture days 5–12). *P<0.05 compared with the 0 ng ml−1BDNF value (analysis of variance with Student Newman–Keulspost-hoctests). (d) Mitochondrial mass determined by mt-green fluorescence intensity normalized to cellular protein concentration (see Methods). (e) Results of measurements of ATP concentrations in hippocampal neurons after 7 days of treatment with BDNF or vehicle; values were normalized to protein concentration. Values are mean±s.d. (n=3 separate cultures). *P<0.05 (Student’st-test). (f) A representative immunoblot of the mitochondrial proteins cox1 and cyt-c, and actin, in neurons that had been treated for 7 days with the indicated concentrations of BDNF. The graph shows the results of densitometric analysis of the blots (n=3 separate cultures). For graphs ind,e,f: *P<0.05, **P<0.01 (Student’st-test). Figure 6: BDNF enhances PGC-1α-mediated mitochondrial biogenesis. ( a , b ) Effects of BDNF on PGC-1α, NRF1 and TFAM mRNA and protein levels in cultured hippocampal neurons. Cultured hippocampal neurons (7 days in culture) were treated with 40 ng ml −1 BDNF for the indicated time periods. mRNA (by quantitative PCR) and protein levels (densitometry analysis) are expressed as fold change compared with the value for vehicle-treated control neurons. Values are mean±s.d. * P <0.05, ** P <0.001 ( n =4; Student’s t -test). ( c ) A representative gel showing mtDNA (left) and results of measurement of the amount of mtDNA normalized to protein concentration in cultured hippocampal neurons after treating with BDNF at indicated concentrations, or vehicle control, for 7 days (from culture days 5–12). * P <0.05 compared with the 0 ng ml −1 BDNF value (analysis of variance with Student Newman–Keuls post-hoc tests). ( d ) Mitochondrial mass determined by mt-green fluorescence intensity normalized to cellular protein concentration (see Methods). ( e ) Results of measurements of ATP concentrations in hippocampal neurons after 7 days of treatment with BDNF or vehicle; values were normalized to protein concentration. Values are mean±s.d. ( n =3 separate cultures). * P <0.05 (Student’s t -test). ( f ) A representative immunoblot of the mitochondrial proteins cox1 and cyt-c, and actin, in neurons that had been treated for 7 days with the indicated concentrations of BDNF. The graph shows the results of densitometric analysis of the blots ( n =3 separate cultures). For graphs in d , e , f : * P <0.05, ** P <0.01 (Student’s t -test). Full size image To determine whether BDNF enhances mitochondrial biogenesis, we treated hippocampal neurons with BDNF or vehicle daily for 7 days beginning on culture day 5, and then measured the amount of mtDNA in the neurons. The mtDNA content of the neurons was significantly increased by approximately twofold in neurons treated with 10–40 ng ml −1 BDNF ( Fig. 6c ). The BDNF-treated (20 ng ml −1 ) neurons exhibited a significant increase (by ~50%) in mitochondrial mass indicated by a greater amount of mt-green fluorescence in BDNF-treated neurons and ATP production (by ~20%) compared with control neurons ( Fig. 6d ). In addition, levels of two mitochondrial proteins, cytochrome oxidase 1 and cyt-c were also elevated considerably in response to BDNF ( Fig. 6f ). PGC-1α mediates BDNF-induced synaptogenesis The findings described above indicated that BDNF signaling significantly increases mitochondrial biogenesis and upregulates PGC-1α expression, and that PGC-1α is important for the development and/or maintenance of dendritic spines and synapses. We next asked whether PGC-1α and PGC-1α-dependent mitochondrial biogenesis mediate BDNF-induced synapse formation. Hippocampal neurons treated with BDNF from culture day 5 until culture day 12 exhibited a significant increase in PSD95-immunoreactive dendritic puncta (84±6.7 puncta per 100 μm dendritic segment; 15–30 neurons analysed, P <0.001, Student’s t -test) compared with control neurons (45±5.3 puncta per 100 μm), whereas the suppression of PGC-1α expression by Ad-si-PGC-1α impaired the ability of BDNF to promote synaptogenesis as indicated by significantly reduced numbers of PSD95-immunoreactive dendritic puncta (52±5.6 puncta per 100 μm dendritic segment; 15–30 neurons analysed, P <0.001 compared with BDNF-treated neurons, Student’s t -test; Fig. 7a ), and abolished the ability of BDNF to increase PSD95 protein levels as determined by immunoblot analysis ( Fig. 7c ). Furthermore, immunoblot analysis showed that the level of BDNF high-affinity receptor TrkB was unchanged in hippocampal neurons with PGC-1α knockdown ( Fig. 7d ). Moreover, immunoprecipitation analysis revealed that phosphorylation of TrkB stimulated by BDNF is unchanged in PGC-1α knockdown neurons compared with either control neurons or Ad-GFP-Si-Con-infected neurons ( Fig. 7e ). Thus, suppression of PGC-1α expression does not affect TrkB levels or its activation by BDNF in hippocampal neurons. These results provide evidence that PGC-1α and PGC-1α-mediated mitochondrial biogenesis serves as a downstream signaling component in the enhancement of synaptogenesis by BDNF. 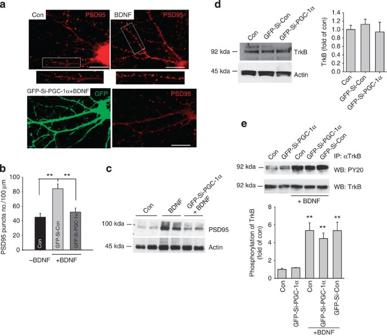Figure 7: PGC-1α knockdown inhibits BDNF-induced synaptogenesis without affecting TrkB expression or activation. (a) Confocal images showing PSD95 immunostaining in cultured hippocampal neurons (12 days in culture) that had been treated with vehicle (Con) or BDNF (40 ng ml−1; BDNF) or transfected with GFP-Si-PGC-1α on culture day 5 and then treated with 40 ng ml−1BDNF (GFP-Si-PGC-1α+BDNF). Scale bar, 20 μm. (b) Results of quantitative analysis of PSD95-immunoreactive puncta in dendrites of neurons from the indicated treatment groups. Bars represent the mean±s.d. (n=5 cultures with 15–30 neurons analysed per condition). **P<0.01 (Student’st-test). (c) Immunoblot analysis of PSD95 protein levels in neurons from the indicated treatment groups. (d) Immunoblot analysis of TrkB in hippocampal neurons 7 days after infection with Ad-GFP-Si-con or Ad-GFP-Si-PGC-1α, compared with uninfected neurons. (e) Immunoprecipitation and quantitative analysis of TrkB physophorylation. TrkB in protein extracts (0.5 mg) from cultured hippocampal neurons in the indicated treatment groups was immunoprecipitated using a rabbit anti-TrkB antibody, and then subjected to immunoblot analysis using the anti-phosphotyrosine antibody PY20 (Cell Signaling Technology). **P<0.01 (n=3; Student’st-test). Figure 7: PGC-1α knockdown inhibits BDNF-induced synaptogenesis without affecting TrkB expression or activation. ( a ) Confocal images showing PSD95 immunostaining in cultured hippocampal neurons (12 days in culture) that had been treated with vehicle (Con) or BDNF (40 ng ml −1 ; BDNF) or transfected with GFP-Si-PGC-1α on culture day 5 and then treated with 40 ng ml −1 BDNF (GFP-Si-PGC-1α+BDNF). Scale bar, 20 μm. ( b ) Results of quantitative analysis of PSD95-immunoreactive puncta in dendrites of neurons from the indicated treatment groups. Bars represent the mean±s.d. ( n =5 cultures with 15–30 neurons analysed per condition). ** P <0.01 (Student’s t -test). ( c ) Immunoblot analysis of PSD95 protein levels in neurons from the indicated treatment groups. ( d ) Immunoblot analysis of TrkB in hippocampal neurons 7 days after infection with Ad-GFP-Si-con or Ad-GFP-Si-PGC-1α, compared with uninfected neurons. ( e ) Immunoprecipitation and quantitative analysis of TrkB physophorylation. TrkB in protein extracts (0.5 mg) from cultured hippocampal neurons in the indicated treatment groups was immunoprecipitated using a rabbit anti-TrkB antibody, and then subjected to immunoblot analysis using the anti-phosphotyrosine antibody PY20 (Cell Signaling Technology). ** P <0.01 ( n =3; Student’s t -test). Full size image Our findings reveal previously unknown roles for PGC-1α in the formation and maintenance of synapses in developing hippocampal neurons, and in the maintenance of synapses in the adult hippocampus. BDNF, which has critical roles in neurogenesis and synaptic plasticity in the developing and adult hippocampus [12] , [13] , [30] , significantly enhanced mitochondrial biogenesis as indicated by increases in mitochondrial mass and upregulation of PGC-1α promoter activity and transcription and expression of PGC-1α, NRF1 and the mitochondrial transcription factor TFAM. Moreover, we found that ERKs and CREB are required for BDNF-induced upregulation of PGC-1α. Mitochondria, as the major energy source in cells, are essential for the excitability and survival of neurons [8] . The formation of hippocampal synapses is associated with increased expression and activation of ligand-gated ion channels and voltage-dependent Ca 2+ channels, which increases the energy demand required to operate the ion-motive ATPases that restore the membrane potential [31] . Mitochondrial biogenesis increases the energy production capability of cells [32] , which may be required for neurons to form and maintain functional synapses. In this study, we selectively modulated mitochondrial biogenesis using molecular genetic methods that target PGC-1α and provided direct evidence that this key regulator of mitochondrial biogenesis also has an important role in the formation of dendritic spines as well as functional synapses. Knockdown of PGC-1α expression, which reduced the amount of mitochondria in dendrites, resulted in decreased density of dendritic spines and synapses. Conversly, overexpression of PGC-1α, which increased mitochondrial biogenesis, also increased levels of synaptic proteins (Synapsin 1 and PSD95). Consistent with a previous report that neurite outgrowth is reduced in cultured striatal neurons from PGC-1α null mice [26] , we found that reduction of PGC-1α levels resulted in a moderate reduction in the complexity of dendritic arbors in embryonic hippocampal neurons. However, knockdown of PGC-1α did not affect dendrite length in adult dentate granule neurons, but did reduce dendritic spine density. These findings suggest that PGC-1α has roles in regulating the dendritic morphology and synaptic connectivity of neuronal circuits in the developing brain, and in the maintenance of synapses in the adult hippocampus. Mitochondrial biogenesis is regulated by several signaling pathways and transcription factors [33] . PGC-1α has been shown previously to induce mitochondrial biogenesis and oxidative metabolism in muscle cells, adipocytes and cardiac myocytes [2] , [3] , [4] . The latter studies also provided evidence that the transcription factor NRF1/2 mediates the effects of PGC-1α on the expression of nuclear genes encoding mitochondrial proteins including the mitochondrial transcription factor (TFAM), which is essential for the initiation of mtDNA transcription and replication [2] , [34] . We found that BDNF significantly enhances PGC-1α, NRF1 and TFAM expression and mitochondrial biogenesis in cultured hippocampal neurons. A functional CRE site in the PGC-1α co-activator gene, which is activated by BDNF-induced activation of ERKs and CREB, mediates PGC-1α expression and mitochondrial biogenesis. Consistent with our findings, previous studies also indicated that CREB activation enhances mitochondrial biogenesis in non-neural cells [34] , [35] . In addition to ERKs, several other kinases regulate CREB activity in neurons including cyclic AMP-dependent protein kinase and calcium/camodulin-dependent kinase [36] , [37] . It is therefore likely that signals that elevate cyclic AMP and Ca 2+ levels will also increase PGC-1α expression and mitochondrial biogenesis in neurons. Binding of BDNF to TrkB results in phosphorylation of tyrosine residues in the cytoplasmic domain of the receptor [38] . Thus activated, TrkB signals via Ras and downstream kinases including mitogen-activated protein kinases and PI3K and Akt kinase [39] , [40] , [41] , [42] . We found that PGC-1α knockdown did not affect levels of TrkB nor its ability to be activated by BDNF, but did significantly reduce the ability of BDNF to increase dendritic spine density. The latter findings suggest PGC-1α has a critical role in mediating the enhancement of synapse formation in response to BDNF. Interestingly, we found that BDNF upregulates PGC-1α in hippocampal neurons by a mechanism involving ERKs and CREB, but not Akt. Previous studies have shown that the PI3K-Akt pathway [43] , ERKs [44] , [45] , [46] and the transcription factor CREB [47] have pivotal roles in synaptic plasticity and learning and memory. Our findings therefore suggest BDNF regulates synapse formation and plasticity by multiple mechanisms, one of which is critically dependent on PGC-1α. Previous studies have shown that several signaling mechanisms that regulate neurite outgrowth also regulate synaptogenesis, with glutamate and BDNF signaling being prominent examples [48] . We found that knockdown of PGC-1α attenuates the ability of BDNF to enhance dendritic spine and synapse formation in embryonic hippocampal neurons. It is therefore likely that PGC-1α has important roles in enabling synaptogenesis as well as neurite outgrowth. Interestingly, as with BDNF, other signaling molecules such as nitric oxide [34] , [49] and estrogen [50] that stimulate PGC-1α and mitochondrial biogenesis in muscle cells also regulate neural plasticity [51] , [52] . In addition, previous studies have shown that exercise and caloric restriction stimulate mitochondrial biogenesis in muscle cells by a PGC-1α-mediated mechanism [2] , [3] , and both exercise and dietary restriction increase BDNF expression [53] , [54] in hippocampus and preserve synaptic function in animal models of Huntington’s [55] , Parkinson’s [56] and Alzheimer’s diseases [57] . Thus, our findings suggest roles for PGC-1α and mitochondrial biogenesis in the protection and plasticity of neuronal circuits throughout life. Reduced levels of PGC-1α have recently been implicated in the pathogenesis of neurodegenerative disorders that involve synaptic degeneration. Studies of animal models and human subjects suggest that in Huntington’s disease mutant huntingtin results in decreased production of cortical BDNF and leads to insufficient neurotrophic support for striatal neurons, which then die [58] . It was recently shown that mutant huntingtin also represses PGC-1α gene transcription by associating with the promoter and interfering with the CREB/TAF4-dependent transcriptional pathway critical for the regulation of PGC-1α gene expression [27] . In addition, selective elimination of PGC-1α in neurons of adult mice results in degeneration of striatal neurons [28] , suggesting that PGC-1α expression may limit the ability of vulnerable neurons to adequately respond to energy demands in Huntington’s disease. Impaired mitochondrial function and deficits in BDNF signaling are also implicated in Alzheimer’s disease [59] , [60] , Parkinson’s disease [55] , [61] and ischemic stroke [62] . It will therefore be of considerable interest to determine whether PGC-1α can be targeted for therapeutic intervention in neurodegenerative disorders. Hippocampal cell cultures and experimental treatments Cultures of hippocampal neurons were prepared from embryonic day 17 Sprague-Dawley rats. Dissociated cells were seeded into polyethyleneimine-coated plastic dishes or glass coverslips in MEM medium supplemented with 10% fetal bovine serum at a density of 30,000 cells cm −2 . After cells attached to the substrate (3 h), the medium was replaced with Neurobasal medium containing B27 supplements (Invitrogen). BDNF was obtained from Invitrogen and PD98059, LY290043 and wortmannin were obtained from Cell Signaling Technology. Immunocytochemistry For immunofluorescence cytochemistry, fixed cells were preincubated with blocking solution (0.2% Triton X-100, 10% normal goat serum) in PBS for 30 min, and then incubated overnight with a primary antibody followed with appropriate secondary antibodies for 2 h at room temperature. The cells were counterstained with propidium iodide or 4′,6-diamidino-2-phenylindole for 10 min. The primary antibodies and their dilutions were as follows: rabbit anti-PGC-1α (1:100, Santa Cruz), anti-synapsin (1:200, Cell Signaling Technology), mouse anti-PSD95 (1:200, Thermo Scientific). The secondary antibody was rhodamine-conjugated goat anti-rabbit (1:500, Molecular Probes). Immunoblot analysis and immunoprecipitation Tissues or cells were solubilized in SDS–PAGE sample buffer, and the protein concentration in each sample was determined using a protein assay kit with bovine serum albumin as the standard. Thirty microgram proteins were resolved on 4–10% SDS polyacrylamide gels and electrophoretically transferred to a nitrocellulose membrane. Following standard methods to incubate the membrane with appropriate primary and secondary antibodies, the reaction product in the membrane was visualized using an ECL Western Blot Detection Kit. The primary antibodies included those that selectively recognize PGC-1α (rabbit, 1:100, Santa Cruz), synapsin 1 (rabbit, 1:1,000, Cell Signaling Technology), synaptophysin (mouse, 1:500, Sigma), Cox1 (mouse, 1:500, Molecular Probes), cytochrome C (mouse, 1:1,000, BD Parmingen), TFAM (rabbit, 1:500, Abcam), NRF1 (rabbit, 1:500, Life Span Bioscience) and, p-CREB,CREB p-AKT, p-ERKs and ERKS (rabbit, 1:1,000, Cell Signaling Technology), PSD95 (mouse, 1:500, Thermo Scientific), actin (mouse, 1:2,000, Sigma). For immunoprecipitation analysis, neurons were solubilized in lysis buffer (150 mM NaCl, 20 mM Tris, pH 7.2, 1.0% Triton X-100, 1% deoxycholate and 5 mM EDTA) with proteinase inhibitor cocktail (Roche Diagnostics, Indianapolis, IN, USA). Equal amounts of protein extracts (0.5 mg) were precleared by incubating with 50 μl of protein A/G agarose (Santa Cruz) for 1 h at 4 °C on a rotating shaker and were then centrifuged to precipitate the beads. Supernatant was collected, incubated with 5 μg of antibodies against TrkB (Santa Cruz, rabbit polyclonal) overnight at 4 °C in a shaker. The samples were then mixed with 100 μl of protein A/G agarose and incubated for 2 h. Pellet protein A/G beads by centrifugation were repeatedly washed four times with 1 ml of lysis buffer, the final pellets were eluted in protein loading buffer, and samples were vortexed and boiled for 3 min. Beads were precipitated by centrifugation, and supernatants were collected for immunoblot analysis using an anti-phosphotyrosine antibody PY20 (Cell Signaling Technology). Quantitative reverse transcriptase PCR amplification Total RNAs were isolated using the RNAeasy purification kit (Qiagen) following manufacturer’s instructions. The complementary DNAs were synthesized using 1 μg total RNA in a 20-μl reaction with Superscript II and oligo(dT)12–18 (Invitrogen). For real-time PCR, the primers and TaqMan probes (for glyceraldehyde-3-phosphate dehydrogenase, PGC-1α, NRF1 and TFAM) and TaqMan Gene Expression Master Mix were purchased from Applied Biosystems. Two microlitre of 20-fold diluted reverse transcription mixture (cDNA) was used as initial template for real-time PCR. The real-time PCR reactions for each RNA sample were performed in triplicate. The default setting of the ABI 7900HT Fast Real-Time PCR System was used for the PCR reaction. The glyceraldehyde-3-phosphate dehydrogenase level was used as the internal control for all other genes. Adenovirus packaging, infections and plasmid transfections Adeno-PGC-1α virus was the generous gift from Dr Pere Puigserver (Johns Hopkins University). Ad-PGC-1α siRNA (GFP-Si-PGC-1α) and Ad-PGC-1α Si-Con (GFP-Si-Con) plasmids, both of which also contain GFP cDNA, were a generous gift from Dr Marc Montminy (The Salk Institute for Biological Studies). The sequence of the PGC RNAi was 5′-GGTGGATTGAAGTGGTGTAGA-3′ (mouse PGC-1α 150–170 bp) and the sequence for the unspecific RNAi control was 5′-GGCATTACAGTATCGAT CAGA-3′. Adeno-PGC-1α virus was amplified by directly infecting HEK293 cells at 70–80% confluence (Invitrogen). Ad-PGC-1α siRNA and Ad-PGC-1α SiCon plasmids were digested with Pac-1, and then were transfected into HEK293 cells to produce adenovirus. Infected or transfected cells were collected and pelleted by centrifugationand high-titer stocks of recombinant adenoviruses were purified by the Adeno-X virus purification kit (Clonetech). The cultured neurons were infected at a multiplicity of infection of 50 p.f.u per cell. To co-transfect mt-DsRed and GFP-Si-PGC-1α or GFP-Si-Con, plasmid DNAs (2 μg each) were mixed and transfected using calcium phosphate in cultured hippocampal neurons. Mitochondrial mass measurements and analysis of mtDNA For mitochondrial mass measurements, cultured hippocampal neurons were loaded with mt-green at final concentration of 500 nM and incubated for 20 min. Equal amounts from each sample lysis were analysed in a Bio Assay Reader (excitation and emission are 485 and 535 nm, respectively, Perkin Elmer) to quantify fluorescence intensity. The values were normalized by protein concentrations. For analysis of mtDNA, mtDNA was isolated from cultured neurons using a Mitochondrial DNA Isolation Kit (Biovison). Briefly, neurons were washed with ice-cold PBS, then scraped and collected in 1 ml cyotsol extraction buffer. After homogenization using a Dounce homogenizer, the homogenates were separated into cytosol (supernatant) and mitochondrial fractions (pellet) by differential centrifugation. The mitochondrial pellets were lysed and incubated in 50 °C in 30 μl of mitochondrial lysis buffer containing protein degradation enzymes. mtDNA was isolated by ethanol precipitation. A small aliqout of homogenates was reserved for protein quantification and mtDNA content were normalized to the protein concentration. Luciferase assay of PGC-1α promoter activity The 2-kb PGC-1α-kb PGC-1 uciferase (PGC-1α-2 kb) and PGC-1α promoter dCRE-luciferase constructs (with a site-directed mutagenesis to remove the CREB-binding site; PGC-1α-ΔCRE) have been described previously [63] . Both constructs were purchased from Addgene. Primary cultured neurons were co-transfected with 2 μg pRL-TK Vector (Promega) expressing Renilla luciferase and 2 μg PGC-1α-2 kb or PGC-1α-ΔCRE using Fugene 6 (Roche) according to the manufacturer’s instructions. Sixteen hours after transfection, cells were incubated in the presence of experimental treatments for 32 h, and luciferase activity was quantified using a Dual-Luciferase-Reporter System (Promega). Luciferase activity in each sample was normalized to the internal control renilla luciferase activity (four to six cultures per condition were analysed). In vivo studies Mice were anesthetized using isoflurane and mounted on a stereotaxic apparatus. A sagittal incision was made through the skin along the midline of the head, and a hole was drilled on the skull at the position of 2.18 mm posterior and 1.6 mm lateral (right) to bregma. The tip of injector was lowered into the dentate gyrus of the hippocampus (1.6 mm below the surface of the brain). One microlitre of solution, containing either Ad-Si-PGC-1α or Ad-GFP-Si-Con (five mice received Ad-GFP-Si-PGC-1α and five mice received Ad-GFP-Si-Con), was injected slowly using a microinjection pump over 3 min. Two weeks after injection, brains were perfusion fixed and processed for immunohistology. Coronal sections containing the dentate gyrus (30 μm thickness) were collected and GFP fluorescence was imaged with a confocal microscope (Zeiss inverted LSM510). FM4-64 labeling Primary hippocampal neurons, which had been transfected with GFP-Si-Con or GFP-Si-PGC-1α, were rinsed with HBSS medium and then incubated 3 min with 5 μM FM4-64FX (Invitrogen) and 100 mM KCl. The cultures were then incubated for 10 min in the presence of the dye without 100 mM KCl to allow for complete endocytosis of all released vesicles. Neurons were then washed with fresh HBSS to remove extracellular FM4-64FX, cells were fixed in 4% paraformaldehyde for 15 min and images of intracellular FM4-64FX fluorescence were acquired using a confocal microscope. Imaging and image analysis For cultured neurons, images were acquired using a Zeiss inverted LSM510 confocal microscope with X63 (numerical aperture (NA), 1.4) or X25 (NA, 0.8) and X10 (NA, 0.3) objectives. The length of dendrites and mitochondria was traced and measured with the aid of LSM510 software. All the spines and dendrites in one image frame were measured. The vast majority of PSD95 or synapsin I puncta were counted along GFP-illustrated dendrites in GFP-Si-PGC-1α− or GFP-Si-Con-transfected neurons. Mitochondrial number in neurites and the dendritic mitochondrial index (total mitochondrial length/dendritic length) were analysed in neurons co-transfected with GFP-Si-PGC-1α or GFP-Si-Con and mt-DsRed. For in vivo analysis of dendritic spine density, segments from secondary and tertiary dendrites on five neurons per mouse were sampled from dentate gyrus region of the hippocampus. Dendritic segments were viewed through a X63 oil immersion objective on a Zeiss confocal microscope. These images were imported into reconstruct for determination of the three-dimensional (3D) length of the segment and spine counting. For analysis of dendritic length and bifurcations, cells were scanned using a X25 objective throughout the apical dendritic arbors. Images stacks were imported into reconstruct for three-dimensional tracing. Statistics All data are presented as mean±s.d. Comparisons between control and treatment groups were performed by using Student’s unpaired t -test or analysis of variance when appropriate. A P -value <0.05 was considered to be statistically significant. How to cite this article: Cheng A. et al . Involvement of PGC-1α in the formation and maintenance of neuronal dendritic spines. Nat. Commun. 3:1250 doi: 10.1038/ncomms2238 (2012).